Formal reply to “Alternative lengthening of telomeres is not synonymous with mutations in ATRX/DAXX” 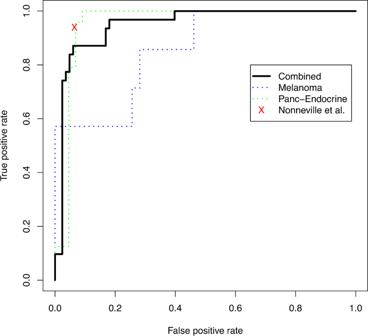Fig. 1: Receiver operating characteristic analysis. The curve shows the True positive rate (sensitivity) and the Fales positive rate (1 – specificity) for all possible thresholds on the ALT probability score (Sieverling et al.1). The predicted class label is the C-circle status reported from Lee et al., while the red cross depicts the performance of the classifier proposed in the Matters Arising article for which classification results are reported for only one threshold. The ROC-curve analysis was conducted with the ROCR package [5] . The ATRX/DAXX trunc score, respectively, ALT probability score from Sieverling et al. [1] was used to evaluate the performance for the individual cohorts and for both cohorts together. As the model in the Matters Arising study does only report a binary classification but no continuous score, the reported performance values of the combined model were marked by a red cross in the diagram. The underlying data is provided as source data in XLSX format. Reporting summary Further information on research design is available in the Nature Research Reporting Summary linked to this article.